Genome-wide associated study identifies NAC42-activated nitrate transporter conferring high nitrogen use efficiency in rice Over-application of nitrogen fertilizer in fields has had a negative impact on both environment and human health. Domesticated rice varieties with high nitrogen use efficiency (NUE) reduce fertilizer for sustainable agriculture. Here, we perform genome-wide association analysis of a diverse rice population displaying extreme nitrogen-related phenotypes over three successive years in the field, and identify an elite haplotype of nitrate transporter OsNPF6.1 HapB that enhances nitrate uptake and confers high NUE by increasing yield under low nitrogen supply. OsNPF6.1 HapB differs in both the protein and promoter element with natural variations, which are differentially trans-activated by OsNAC42, a NUE-related transcription factor. The rare natural allele OsNPF6.1 HapB , derived from variation in wild rice and selected for enhancing both NUE and yield, has been lost in 90.3% of rice varieties due to the increased application of fertilizer. Our discovery highlights this NAC42-NPF6.1 signaling cascade as a strategy for high NUE and yield breeding in rice. Application of nitrogen fertilizer has been a routine way to sustain crop productivity. There is increasing interest in using nitrogen use efficiency (NUE) genes to breed high-NUE cultivars due to the unnecessary costs to farmers and the deleterious impact on the environment caused by increased use of nitrogen fertilizers [1] , [2] . However, plant NUE is inherently complex, since it involves nitrogen (N) sensing, uptake, translocation, assimilation, and remobilization, and is governed by multiple interacting genetic and environmental factors [3] , [4] , [5] . Enhanced N acquisition must be accompanied by efficient transport and assimilation to drive growth and development, including increased plant height (PH), effective panicle number (EPN) and yield per plant (YPP) [6] . Increasing our knowledge of genes and interactions associated with these critical processes will accelerate the breeding of NUE. Rice ( Oryza sativa L.) is a major crop, feeding almost 50% of the world’s population. Most attempts to identify NUE-related traits have focused on quantitative trait locus (QTL) mapping using bi-parental populations. Major NUE genes have been identified including nitrate-transporter genes OsNRT1.1A , OsNRT1.1B , OsNRT2.3 [7] , [8] , [9] and transcription factor OsGRF4 [10] . Changes in the amino acid sequences of nitrate transporters of yeast Hansenula polymorpha (Ynt1), Arabidopsis thaliana (AtCHL1/AtNPF6.3/AtNRT1.1), and Oryza sativa (OsNRT1.1B) have been reported to influence their transport activities [8] , [11] , [12] . However, variation in alleles that cause NUE differences between diverse rice varieties, has not been intensively explored. Compared to traditional bi-parental linkage analysis, association mapping has the potential to identify QTLs in a core population consisting of hundreds of landraces, with the power to detect simultaneously multiple loci with multiple alleles at a locus [13] , [14] , [15] , [16] . Association mapping is a high-resolution method for dissecting complex genetic traits in plants. Extreme-phenotype genome-wide associated study (GWAS), has been proposed as an approach that does not require genotyping large numbers of individuals. Instead, it relies on genotyping individuals from a diverse panel that has extreme phenotypes [17] . We previously evaluated genetic diversity and breeding values of these varieties for rice NUE [18] , and identified polymorphic single nucleotide polymorphisms (SNPs) through genotyping by sequencing [19] . However, very few studies have taken advantage of GWAS to examine core populations through field experiments for identification of natural variations in alleles and regulatory networks promoting crop NUE. Here, we carry out GWAS with a population consisting of rice landraces with extreme N-related phenotypes. We identify seven NUE-related genes and prioritize two genes, OsNPF6.1 and OsNAC42 , for functional analyses. We show that, out of the ordinary nitrate transporters in yeasts and plants, OsNPF6.1 alleles differ in both protein and promoter element sequences. OsNPF6.1 HapB is transactivated by transcription factor OsNAC42, and enhances NUE by increasing EPN and yield. Identification and functional validation of OsNPF6.1 HapB We measured the NUE-related agronomic traits of PH, EPN, and YPP of the 117 studied lines with extreme N-related phenotypes grown in low nitrogen (LN) and high nitrogen (HN) fields in the years 2014–2016 (Supplementary Fig. 1a ). The trait values obviously decreased under LN treatment, so the LN treatment was proved to be effective (Supplementary Fig. 1b ). To reflect NUE, we focused on trait ratios (the ratio of the trait value under LN to the trait value under HN). 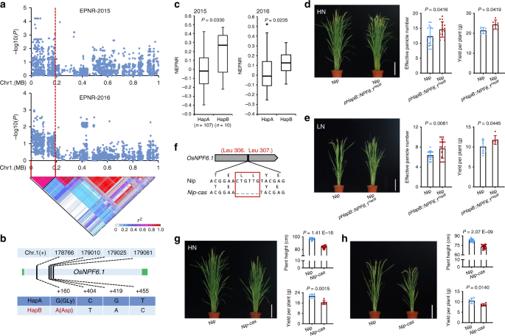Fig. 1 Identification and functional validation ofOsNPF6.1on chromosome 1.aLocal Manhattan plot (top) and LD heatmap (bottom) surrounding the peak on chromosome 1. Red dashed line indicates the candidate region for the peak.bGene structure ofOsNPF6.1and DNA polymorphism in this gene. Green boxes and light blue box represent UTR and exon, respectively.cComparative analyses ofOsNPF6.1between the low and high NUE haplotypes. NEPNR (normalized effective panicle number ratio)-2015 (left) and NEPNR-2016 (right) based on the haplotypes (Hap) ofOsNPF6.1. Box edges represent the 0.25 quantile and 0.75 quantile with the median values shown by bold lines. Whiskers extend to data no more than 1.5 times the interquartile range, and remaining data are indicated by dots. Differences between the haplotypes were analyzed by Welch’sttest.d,eComparison of the effective panicle numbers and yields per plant of Nip and complementary line (NippHapB::NPF6.1HapB) in HN and LN, bar = 20 cm,n= 16, 6.fTwo amino acids are deleted inNip-cas. Red box indicates the missing amino acids.g,hComparison of Nip and knock-out line (Nip-cas) plant heights and yields per plant under HN and LN conditions, bar = 20 cm,n= 16, 6. Data are presented as means ± SD.Pvalues (versus the Nip) were calculated with Student’sttest. Nip Nipponbare. The source data underlying Figs.1d, e, g, andhare provided as a Source Data file. PH ratio (PHR), EPN ratio (EPNR), and YPP ratio (YPPR) were then calculated for each line in each year (Supplementary Table 1 , Supplementary Fig. 1c ). Through observing the NUE-associated phenotypes, we found that the cultivars Nanjing11 and JC92 were hyposensitive to LN treatment since the NUE-associated phenotypes of Nanjing11 and JC92 under LN treatment were similar to those under HN treatment. On the other hand, the cultivars Samchun and Shannong13 displayed high sensitivity to LN treatment as the NUE-associated phenotypes were significantly weaker under LN treatment. The ratios were significantly different between the hyposensitive and sensitive varieties (Supplementary Fig. 3a ). We performed GWAS on NUE-related agronomic traits to identify statistically associated genes (Supplementary Figs. 2 , 3 and Supplementary Data 1 , see Supplementary Notes 1 and 2 ). 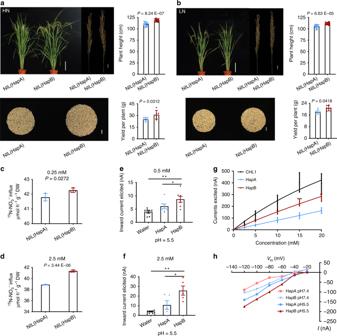Fig. 2 Functional analysis of OsNPF6.1.a,bComparison of the plant heights and yields per plant of NIL (HapA) and NIL (HapB), under HN (a) and LN (b) conditions, bar = 20 cm (the plants), 2 cm (the panicles and the seeds),n= 16, 6.c,dNitrate influx rates in the roots. The root nitrate influx was measured in 0.25 mM (c) or 2.5 mM (d)15NO3−,n= 3. Data are presented as means ± SD.Pvalues were calculated with Student’sttest.e,fAverages of the currents elicited under 0.5 mM (e) and 2.5 mM NO3−(f) in oocytes injected with complementary RNAs of the coding regions of two haplotypes (OsNPF6.1HapAandOsNPF6.1HapB) ofOsNPF6.1or water control. The oocytes were voltage-clamped at −60 mV, and the inward currents elicited with 0.5 mM or 2.5 mM NO3−at pH 5.5. Bars represent mean ± SEM,n= 7 (e),n= 7, 5, 5 (f). One-way analysis of variance (ANOVA) followed by Tukey’s multiple comparison test was used to analyze statistical significance (*P< 0.05 and **P< 0.01).gConcentration dependence of nitrate-elicited currents in a single injected oocyte. The oocyte was voltage-clamped at −60 mV, and the currents elicited by different concentrations of nitrate (0–20 mM) at pH 5.5, AtCHL1 as a positive control. Each bar represents the mean ± SEM,n= 4, 10, 10 (*P< 0.05 and **P< 0.01, Welch’sttest).hCurrent-to-voltage relationship forOsNPF6.1HapAandOsNPF6.1HapB. The curves presented were recorded from a singleOsNPF6.1HapA(blue) andOsNPF6.1HapB(red)-injected oocyte treated with 10 mM nitrate at pH 5.5, andOsNPF6.1HapA(light red) andOsNPF6.1HapB(light blue) all at 10 mM and pH 7.4. The data in (e–h) obtained from independent oocytes from the same frog, and similar results were obtained from three different frogs. Source data are provided as a Source Data file. Seven SNP loci associated with NUE-related traits were repeatedly detected on chromosomes 1, 2, 3, 9, 10, and 12 (Supplementary Table 2 and Supplementary Fig. 3b ). Literature queries showed that five previously reported NUE-related genes were detected in this study, including OsNPF2.4 and OsNRT1.1B which are involved in N transport, and OsNiR and OsGS1;1 which are involved in N assimilation (Supplementary Table 2 ). We identified two loci located on chromosomes 1 and 9 (Supplementary Table 2 and Supplementary Fig. 3c ). The two loci, which we designated EPNR-1 and PHR-9 , were investigated using local LD analysis to identify the NUE-related genes which they harbored (see Supplementary Note 3 ). On chromosome 1, the candidate gene of EPNR-1 was predicted to reside in the region spanning bp 0–190,786 (Fig. 1a ), containing 112 gene-localized SNPs (Fig. 1a ). Through SNP annotation analysis, missense-variant SNP polymorphisms were detected in eight genes (Supplementary Fig. 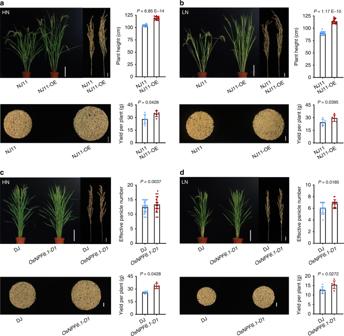Fig. 3 Agronomic traits enhanced by ectopic expression ofOsNPF6.1.a,bComparison of NJ11 and NJ11-OE plant heights under HN (a) and LN (b) conditions, bar = 20 cm (the plants), 2 cm (the panicles and the seeds),n= 16, 6.c,dComparison of the effective panicle numbers at maturity of DJ andOsNPF6.1-D1in HN (c) and LN (d) conditions, bar = 20 cm (the plants), 2 cm (the panicles and the seeds),n= 16, 5. Data are presented as means ± SD.Pvalues (versus the NJ11 and DJ) were calculated with Student’sttest. NJ11, Nanjing11; DJ, Dongjin. Source data are provided as a Source Data file. 4a , Supplementary Table 3 ). By gene-expression analyses, we found that Os01g0103100 , which encodes a nitrogen transporter OsNPF6.1 belonging to the NRT1/PTR family (NPF) [20] , was transcriptionally induced by nitrate application (Supplementary Fig. 4b ). Intriguingly, the two OsNPF6.1 haplotypes contained four SNPs in the core population (Fig. 1b ), and showed differences in EPNR (Fig. 1c ). Fig. 1 Identification and functional validation of OsNPF6.1 on chromosome 1. a Local Manhattan plot (top) and LD heatmap (bottom) surrounding the peak on chromosome 1. Red dashed line indicates the candidate region for the peak. b Gene structure of OsNPF6.1 and DNA polymorphism in this gene. Green boxes and light blue box represent UTR and exon, respectively. c Comparative analyses of OsNPF6.1 between the low and high NUE haplotypes. NEPNR (normalized effective panicle number ratio)-2015 (left) and NEPNR-2016 (right) based on the haplotypes (Hap) of OsNPF6.1 . Box edges represent the 0.25 quantile and 0.75 quantile with the median values shown by bold lines. Whiskers extend to data no more than 1.5 times the interquartile range, and remaining data are indicated by dots. Differences between the haplotypes were analyzed by Welch’s t test. d , e Comparison of the effective panicle numbers and yields per plant of Nip and complementary line (Nip pHapB::NPF6.1 HapB ) in HN and LN, bar = 20 cm, n = 16, 6. f Two amino acids are deleted in Nip-cas . Red box indicates the missing amino acids. g , h Comparison of Nip and knock-out line ( Nip-cas ) plant heights and yields per plant under HN and LN conditions, bar = 20 cm, n = 16, 6. Data are presented as means ± SD. P values (versus the Nip) were calculated with Student’s t test. Nip Nipponbare. The source data underlying Figs. 1 d, e, g, and h are provided as a Source Data file. Full size image To further study the role of OsNPF6.1 HapB in NUE, we introduced OsNPF6.1 HapB into Nip (Nipponbare) under the control of its native promoter, and compared EPN and YPP of Nip with those of the complementary line (Fig. 1d, e ). As expected, both EPN and YPP of Nip pHapB::NPF6.1 HapB were significantly increased compared to those of Nip ( OsNPF6.1 HapA ) (Fig. 1d, e ). We constructed knock-out line ( Nip-cas ) of Nipponbare ( OsNPF6.1 HapA ) by using the CRISPR/Cas system (Fig. 1f ). The agronomic traits of PH and YPP were significantly reduced in Nip-cas as compared to Nip, under either HN or LN conditions (Fig. 1g, h ). These data suggest an important role of OsNPF6.1 in regulating NUE. Physiological functions of OsNPF6.1 HapB To validate the difference between the two haplotypes, we determined the phenotypes and OsNPF6.1 gene-expression levels in near-isogenic lines (NILs) with 415 kb substitution segments containing HapA or HapB of OsNPF6.1 (Supplementary Fig. 5a ). In terms of PH and YPP, NIL (HapB) performed better than NIL (HapA) under both HN and LN conditions (Fig. 2a, b ). Accordingly, higher expression of OsNPF6.1 was detected in NIL (HapB) than in NIL (HapA), especially under LN condition (Supplementary Fig. 5b ). 15 N-nitrate uptake assay also showed that more nitrate was detected in NIL (HapB) than NIL (HapA) when supplied with both low and high concentrations of 15 N-nitrate (Fig. 2c, d ). Fig. 2 Functional analysis of OsNPF6.1. a , b Comparison of the plant heights and yields per plant of NIL (HapA) and NIL (HapB), under HN ( a ) and LN ( b ) conditions, bar = 20 cm (the plants), 2 cm (the panicles and the seeds), n = 16, 6. c , d Nitrate influx rates in the roots. The root nitrate influx was measured in 0.25 mM ( c ) or 2.5 mM ( d ) 15 NO 3 − , n = 3. Data are presented as means ± SD. P values were calculated with Student’s t test. e , f Averages of the currents elicited under 0.5 mM ( e ) and 2.5 mM NO 3 − ( f ) in oocytes injected with complementary RNAs of the coding regions of two haplotypes ( OsNPF6.1 HapA and OsNPF6.1 HapB ) of OsNPF6.1 or water control. The oocytes were voltage-clamped at −60 mV, and the inward currents elicited with 0.5 mM or 2.5 mM NO 3 − at pH 5.5. Bars represent mean ± SEM, n = 7 ( e ), n = 7, 5, 5 ( f ). One-way analysis of variance (ANOVA) followed by Tukey’s multiple comparison test was used to analyze statistical significance (* P < 0.05 and ** P < 0.01). g Concentration dependence of nitrate-elicited currents in a single injected oocyte. The oocyte was voltage-clamped at −60 mV, and the currents elicited by different concentrations of nitrate (0–20 mM) at pH 5.5, AtCHL1 as a positive control. Each bar represents the mean ± SEM, n = 4, 10, 10 (* P < 0.05 and ** P < 0.01, Welch’s t test). h Current-to-voltage relationship for OsNPF6.1 HapA and OsNPF6.1 HapB . The curves presented were recorded from a single OsNPF6.1 HapA (blue) and OsNPF6.1 HapB (red)-injected oocyte treated with 10 mM nitrate at pH 5.5, and OsNPF6.1 HapA (light red) and OsNPF6.1 HapB (light blue) all at 10 mM and pH 7.4. The data in ( e – h ) obtained from independent oocytes from the same frog, and similar results were obtained from three different frogs. Source data are provided as a Source Data file. Full size image Compared with the crystal structure of AtCHL1 [20] , the predicted secondary structure of OsNPF6.1 contains 12 transmembrane (TM)-spanning alpha helices (Supplementary Fig. 6 ). The amino-terminal and carboxyl-terminal domains are cytoplasmic and a long extracellular domain extends outwards from the transporter domain. In rice protoplasts, OsNPF6.1-GFP (green fluorescent protein) fusion proteins are localized to the plasma membrane (PM) since it co-localizes with the PM-OsSCAMP1 (Supplementary Fig. 7a ) [21] , [22] . These results imply that PM-localized OsNPF6.1 might directly transport nitrate. We examined the β-glucuronidase (GUS) activity of OsNPF6.1Pro:GUS transgenic line and found that OsNPF6.1 expressed highly in the rice root tissues (Supplementary Fig. 8a–f ), including lateral roots (Supplementary Fig. 8f ) and epidermal cells of rice root (Supplementary Fig. 8c ). In addition to root, we also observed its expression on rice lamina joint (Supplementary Fig. 8g, h ), so we believed that OsNPF6.1 played roles in direct uptake and redistribution of nitrate. We next examined whether OsNPF6.1 HapA and OsNPF6.1 HapB encoded a functional nitrate transporter by using the Xenopus laevis oocyte heterologous expression system. When voltage was clamped at −60 mV, we found that under concentrations of NO 3 − (0.5 and 2.5 mM), oocytes expressing OsNPF6.1 HapA and OsNPF6.1 HapB both showed higher nitrate uptake compared to water-injected controls, and higher nitrate uptakes were detected in oocytes expressing OsNPF6.1 HapB (Fig. 2e, f ). These results indicated that OsNPF6.1 has nitrate transport activity, and OsNPF6.1 HapB responded to nitrate more strongly than OsNPF6.1 HapA at the same NO 3 − concentration. We previously showed a higher nitrate uptake by NIL (HapB) as compared to (HapA) (Fig. 2c, d ), therefore the difference in nitrate affinity between OsNPF6.1 HapA and OsNPF6.1 HapB was determined. Both OsNPF6.1 HapA and OsNPF6.1 HapB -injected oocytes were exposed to varying concentrations of nitrate (0–20 mM) at pH 5.5 and AtCHL1 was used as a positive control. The amplitudes of the inward currents elicited by nitrate at pH 5.5 were concentration-dependent. A significant leftward shift was observed in the dose–dependent response of OsNPF6.1 HapB to NO 3 − as compared to OsNPF6.1 HapA (Fig. 2g , Supplementary Fig. 9 ). The elicited current differed between OsNPF6.1 HapA and OsNPF6.1 HapB -injected oocytes at all membrane potentials tested from −120 to −20 mV (Fig. 2h ). Under the same concentration of NO 3 − , the amplitudes of the inward currents elicited by exposure to nitrate were pH-dependent in both OsNPF6.1 HapA and OsNPF6.1 HapB -injected oocytes, being larger at pH 5.5 than at pH 7.4 in both haplotypes. Meanwhile, the average amplitudes of the inward currents of OsNPF6.1 HapB -injected oocytes were larger than OsNPF6.1 HapA -injected oocytes at the same pH (Fig. 2h ). These results collectively reveal that OsNPF6.1 HapB is the elite haplotype that enhances NUE by increasing N uptake. Transcriptional regulation of OsNPF6.1 is critical for NUE Expression of OsNPF6.1 corresponds with EPN under HN and LN conditions with correlation coefficients of 0.61 and 0.81 respectively (Supplementary Fig. 10a ). Overexpression of OsNPF6.1 HapA in Nip promoted EPN and YPP in HN and LN fields as compared to wild-type Nip (Supplementary Fig. 10b–d ). These results collectively suggested that HapB was a superior haplotype for NUE. As OsNPF6.1 HapB was superior to OsNPF6.1 HapA at nitrogen uptake, we further constructed overexpression lines (NJ11-OE) of NJ11 (Nanjing11, OsNPF6.1 HapB ) (Supplementary Fig. 10e ), and detected increased PH and YPP in these lines under either HN or LN conditions (Fig. 3a, b ). This confirmed that the transcriptional level of OsNPF6.1 is critical for NUE-related traits. Fig. 3 Agronomic traits enhanced by ectopic expression of OsNPF6.1 . a , b Comparison of NJ11 and NJ11-OE plant heights under HN ( a ) and LN ( b ) conditions, bar = 20 cm (the plants), 2 cm (the panicles and the seeds), n = 16, 6. c , d Comparison of the effective panicle numbers at maturity of DJ and OsNPF6.1-D1 in HN ( c ) and LN ( d ) conditions, bar = 20 cm (the plants), 2 cm (the panicles and the seeds), n = 16, 5. Data are presented as means ± SD. P values (versus the NJ11 and DJ) were calculated with Student’s t test. NJ11, Nanjing11; DJ, Dongjin. Source data are provided as a Source Data file. Full size image Meanwhile, the ratios of N concentrations under LN and HN (LN/HN) were increased in flag, secondary and other leaves of NIL (HapB), OsNPF6.1-D1 (4A-03841L, a gain-of-function T-DNA insertion line in the Dongjin background), Nip complementary line and Nip lines over-expressing OsNPF6.1 , compared to those of NIL (HapA), Dongjin, and Nip, respectively (Supplementary Fig. 11a–c ). We measured the nitrogen and nitrate concentration in tillering node of Nip and the complementary line. The results showed that the nitrogen concentration and nitrate concentration of the complementary line were both higher than Nip. We further measured the nitrogen and nitrate concentration in tillering node of Nip lines over-expressing OsNPF6.1 . The results showed that the nitrogen concentration and nitrate concentration of Nip lines over-expressing OsNPF6.1 higher than Nip except for OsNPF6.1OE-6 or OsNPF6.1OE-12 (Supplementary Fig. 11d ). These results strongly suggest a positive correlation between OsNPF6.1 transcriptional level and N concentration in vivo. Remarkably, in the OsNPF6.1-D1 gain-of-function mutant, the T-DNA insertion was detected in the promoter region of OsNPF6.1 (Supplementary Fig. 12a, b ), indicating that the OsNPF6.1 -promoter is critical to regulate its expression for proper nitrate uptake and NUE-traits (Fig. 3c, d ). We observed that all OsNPF6.1 HapB accessions had identical promoter sequences with 73 SNPs and 14 Indels, but different transcription factor binding sites compared to OsNPF6.1 HapA (Supplementary Fig. 13a, b ). We further found that two additional CACG motifs contribute to higher expression levels (Supplementary Fig. 13c ). This implied that the haplotypes of OsNPF6.1 are probably regulated differently at the transcriptional level. OsNAC42 binds and activates the promoters of OsNPF6.1 HapB To identify a possible OsNPF6.1 transcriptional regulator, we searched possible loci which encoded transcription factors. From our GWAS, we also identified a NUE-associated locus that was predicted to reside between bp 18,387,845 and 19,167,561 of chromosome 9. It included 335 SNPs, and contained missense mutations in 16 genes (Fig. 4a , Supplementary Fig. 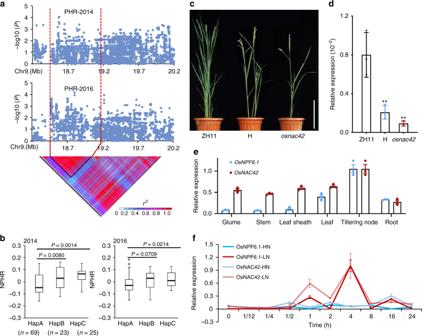Fig. 4 Identification and functional validation of the transcription factorOsNAC42on chromosome 9.aLocal Manhattan plot (top) and LD heatmap (bottom) surrounding the peak on chromosome 9. Red dashed lines indicate the candidate region for the peak.bComparative analyses ofOsNAC42between the low and high NUE haplotypes. Boxplots for NPHR (normalized plant height ratio)-2014 (top) and NPHR-2016 (bottom) based on the haplotypes (Hap) forOsNAC42. Box edges represent the 0.25 quantile and 0.75 quantile with the median values shown by bold lines. Whiskers extend to data no more than 1.5 times the interquartile range, and remaining data are indicated by dots. Differences between the haplotypes were analyzed by Welch’sttest.cPhenotype of WT (Zhonghua11, ZH11), Tilling mutant (osnac42) and heterozygote (H), bar = 20 cm.dqRT-PCR analysis ofOsNPF6.1of WT (Zhonghua11, ZH11), Tilling mutant (osnac42) and heterozygote (H). Three biological replicates were used for qRT-PCR.eOsNPF6.1andOsNAC42transcript levels in different tissues.OsActin1was used as a control,n= 3.fOsNPF6.1andOsNAC42expression under HN treatment from 0 to 24 h in leaf (KCl as a control of LN representing nitrogen starvation),n= 3. Data are presented as means ± SD.Pvalues (versus the ZH11) were calculated with Student’sttest. **P< 0.01. The source data underlying Fig.4d–fare provided as a Source Data file. 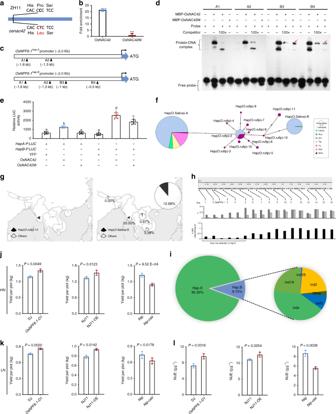Fig. 5 OsNPF6.1HapBstably transactivated by OsNAC42 and rarely utilized in NUE improvement.aSchematic diagram ofOsNAC42tilling mutant (osnac42). ZH11, Zhonghua11.bChIP assays by OsNAC42 and OsNAC42M on binding with DNA of the promoter region ofOsNPF6.1HapA. The fold enrichment was normalized against riceubiquitinpromoter,n= 3. Each bar represents the mean and SEM. **P< 0.01.cSchematic diagram of promoter haplotypes ofOsNPF6.1(OsNPF6.1HapAandOsNPF6.1HapB). The black triangles represent CACG motifs. Four CACG motif regions (A1, A2, B3, and B4) under triangles indicate the positions of the probes used in EMSA assays.dDNA binding activities of OsNAC42 and OsNAC42 mutant proteins on four CACG motif regions of theOsNPF6.1HapAandOsNPF6.1HapBpromoters were tested by EMSA. Red arrows highlight B3 and B4 binding sites. (e) Transactivation activities of OsNAC42 and OsNAC42 mutant (OsNAC42M) on promoter of twoOsNPF6.1haplotypes(HapA-PandHapB-P). YFP, OsNAC42, and OsNAC42M proteins were used as effectors,n= 8.P< 0.05.fHaplotype network of theOsNPF6.1 gene. Each haplotype is separated by mutational changes, with hatches indicating differences between linked haplotypes.aro,aromatic;tej,temperate japonica;trj,tropical japonica;adx,admix;wild,O. rufipogon.gGeographical distribution of theOsNPF6.1inO. rufipogonandO. sativa. The pie chart size is proportional to the number of accessions.hNucleotide diversity across theOsNPF6.1genomic region. Top: The 17 sampled loci (includingOsNPF6.1) located in the genomic region around theOsNPF6.1gene on chromosome 1. Middle: Nucleotide diversitypiof Hap X and B rice at the sampled loci.iTotally, 209 varieties harboringOsNPF6.1HapB, accounting for only 9.7% with 97.3% inindica.j, kYield per plot ofOsNPF6.1-D1,OsNPF6.1HapBoverexpression line andOsNPF6.1HapAknock-out line in HN and LN fields,n= 3.lNUE (grain yield—grain yield of zero-N plot (6 × 8)/N supply) ofOsNPF6.1-D1,OsNPF6.1HapBoverexpression line andOsNPF6.1HapAknock-out line,n= 3. Data are presented as means ± SD. DJ, Dongjin; NJ11, Nanjing11; Nip, Nipponbare. The source data underlying Fig.5b, d, e, h, j–lare provided as a Source Data file. 14 , Supplementary Table 4 ). Among them, a NAC (NAM/ATAF1/2/CUC2) family transcriptional factor gene OsNAC42 was upregulated by LN (Supplementary Fig. 15 ). Agreeing with the hypothesis of possible genetic interaction between OsNAC42 and OsNPF6.1 , both of them were highly expressed in leaf (Fig. 4e ). Expressions of the two genes reached a peak in leaf at 4 h post N starve treatment (Fig. 4f ). Three haplotypes of OsNAC42 were identified based on polymorphism of the promoter. Among them, OsNAC42 HapC was found to be the elite allele as it showed higher PHR levels and expression levels than either OsNAC42 HapA or OsNAC42 HapB (Fig. 4b , Supplementary Fig. 16 ). By contrast, PH and EPN were substantially decreased in the homozygous and heterozygous lines of an osnac42 tilling mutant (Fig. 4c ), which carries a lost-of-function SNP mutation (Pro51 changed to Leu, P51L) (Fig. 5a ). Fig. 4 Identification and functional validation of the transcription factor OsNAC42 on chromosome 9. a Local Manhattan plot (top) and LD heatmap (bottom) surrounding the peak on chromosome 9. Red dashed lines indicate the candidate region for the peak. b Comparative analyses of OsNAC42 between the low and high NUE haplotypes. Boxplots for NPHR (normalized plant height ratio)-2014 (top) and NPHR-2016 (bottom) based on the haplotypes (Hap) for OsNAC42 . Box edges represent the 0.25 quantile and 0.75 quantile with the median values shown by bold lines. Whiskers extend to data no more than 1.5 times the interquartile range, and remaining data are indicated by dots. Differences between the haplotypes were analyzed by Welch’s t test. c Phenotype of WT (Zhonghua11, ZH11), Tilling mutant ( osnac42 ) and heterozygote (H), bar = 20 cm. d qRT-PCR analysis of OsNPF6.1 of WT (Zhonghua11, ZH11), Tilling mutant ( osnac42 ) and heterozygote (H). Three biological replicates were used for qRT-PCR. e OsNPF6.1 and OsNAC42 transcript levels in different tissues. OsActin1 was used as a control, n = 3. f OsNPF6.1 and OsNAC42 expression under HN treatment from 0 to 24 h in leaf (KCl as a control of LN representing nitrogen starvation), n = 3. Data are presented as means ± SD. P values (versus the ZH11) were calculated with Student’s t test. ** P < 0.01. The source data underlying Fig. 4 d– f are provided as a Source Data file. Full size image Fig. 5 OsNPF6.1 HapB stably transactivated by OsNAC42 and rarely utilized in NUE improvement. a Schematic diagram of OsNAC42 tilling mutant ( osnac42 ). ZH11, Zhonghua11. b ChIP assays by OsNAC42 and OsNAC42M on binding with DNA of the promoter region of OsNPF6.1 HapA . The fold enrichment was normalized against rice ubiquitin promoter, n = 3. Each bar represents the mean and SEM. ** P < 0.01. c Schematic diagram of promoter haplotypes of OsNPF6.1 ( OsNPF6.1 HapA and OsNPF6.1 HapB ). The black triangles represent CACG motifs. Four CACG motif regions (A1, A2, B3, and B4) under triangles indicate the positions of the probes used in EMSA assays. d DNA binding activities of OsNAC42 and OsNAC42 mutant proteins on four CACG motif regions of the OsNPF6.1 HapA and OsNPF6.1 HapB promoters were tested by EMSA. Red arrows highlight B3 and B4 binding sites. ( e ) Transactivation activities of OsNAC42 and OsNAC42 mutant (OsNAC42M) on promoter of two OsNPF6.1 haplotypes (HapA-P and HapB-P) . YFP, OsNAC42, and OsNAC42M proteins were used as effectors, n = 8. P < 0.05. f Haplotype network of the OsNPF6. 1 gene. Each haplotype is separated by mutational changes, with hatches indicating differences between linked haplotypes. aro , aromatic ; tej , temperate japonica ; trj , tropical japonica ; adx , admix ; wild , O. rufipogon . g Geographical distribution of the OsNPF6.1 in O. rufipogon and O. sativa . The pie chart size is proportional to the number of accessions. h Nucleotide diversity across the OsNPF6.1 genomic region. Top: The 17 sampled loci (including OsNPF6.1 ) located in the genomic region around the OsNPF6.1 gene on chromosome 1. Middle: Nucleotide diversity pi of Hap X and B rice at the sampled loci. i Totally, 209 varieties harboring OsNPF6.1 HapB , accounting for only 9.7% with 97.3% in indica . j, k Yield per plot of OsNPF6.1-D1 , OsNPF6.1 HapB overexpression line and OsNPF6.1 HapA knock-out line in HN and LN fields, n = 3. l NUE (grain yield—grain yield of zero-N plot (6 × 8)/N supply) of OsNPF6.1-D1 , OsNPF6.1 HapB overexpression line and OsNPF6.1 HapA knock - out line, n = 3. Data are presented as means ± SD. DJ, Dongjin; NJ11, Nanjing11; Nip, Nipponbare. The source data underlying Fig. 5 b, d, e, h, j– l are provided as a Source Data file. Full size image Interestingly, Pro51 is a highly conserved amino acid in the NAC transcription factor family and is involved in binding to the promoters of the genes they regulate [23] . In the osnac42 mutant, the expression of OsNPF6.1 was dramatically decreased (Fig. 4d ), thus OsNPF6.1 expression might be transactivated by OsNAC42. Meanwhile, OsNAC42 localizes to the nucleus, consistent with its function as a transcriptional factor (Supplementary Fig. 7b ). We measured lower nitrate influx rate in the osnac42 mutant under 0.25 mM NO 3 − treatment for 1 h (Supplementary Fig. 17a ). We also measured the nitrogen concentration in tillering node of ZH11 and osnac42 mutant. The result showed that the nitrogen concentration of osnac42 mutant was lower than ZH11 (Supplementary Fig. 17b ). To clarify the potential genetic interactions between OsNPF6.1 and OsNAC42 , we first performed chromatin immunoprecipitation (ChIP)-polymerase chain reaction (PCR) and confirmed in vivo association of OsNAC42 with CACG-containing promoter fragments from OsNPF6.1 (Fig. 5b ). The CACG motif is a well-characterized binding site of NAC transcription factors [24] , and there are two more CACG motifs (B3 and B4) in the promoter region of OsNPF6.1 HapB than in that of OsNPF6.1 HapA (Fig. 5c ). We next tested whether OsNAC42 protein could bind the OsNPF6.1 promoter elements by performing electrophoretic mobility shift assays (EMSA) with purified WT OsNAC42 and mutated OsNAC42 (OsNAC42M, P51L, protein encoded in osnac42 tilling mutant) proteins. Our results showed that OsNAC42 protein was capable of binding to CACG motifs in the promoters of OsNPF6.1 HapA and OsNPF6.1 HapB (Fig. 5d ), whereas OsNAC42M protein could only bind the CACG sites of OsNPF6.1 HapB in the B3 and B4 regions of the promoter (Fig. 5d ). We next tested the ability of OsNAC42 protein and the corresponding mutated version to drive expression of the OsNPF6.1 HapA and OsNPF6.1 HapB promoters, which were fused to the luciferase gene and co-introduced into Nicotiana benthamiana leaves with constructs driving the expression of OsNAC42 or osnac42 (C 19124794 changed to T, identical to the mutation in osnac42 tilling mutant) (Supplementary Fig. 18a ). Luciferase activity driven by either promoter was highly enhanced in the presence of OsNAC42 (Fig. 5e ), suggesting that OsNAC42 could trans-activate OsNPF6.1 expression, especially of OsNPF6.1 HapB . On the other hand, the mutated version of OsNAC42 (OsNAC42M) failed to trans-activate the OsNPF6.1 HapA promoter (Fig. 5e ), but increased the activation level of OsNPF6.1 HapB , though the activity was less than that of WT OsNAC42, suggesting that OsNPF6.1 HapB is more sensitive to OsNAC42 and tolerates NAC variation. Therefore, OsNAC42 is a crucial regulator of the transcriptional activation of OsNPF6.1 , especially OsNPF6.1 HapB . Potential breeding utilization of OsNPF6.1 HapB We investigated OsNPF6.1 presence in a wild ancestor of cultivated rice O. sativa , Oryza rufipogon . Gene haplotype network analysis showed that wild and cultivated rice shared OsNPF6.1 HapA , while OsNPF6.1 HapB emerged in O. rufipogon during Hap( O. rufipogon )-12 differentiation (Fig. 5f ). Hap( O. rufipogon )-12 originated from Myanmar (Fig. 5g left) and then OsNPF6.1 HapB might be a target of selection for the cultivation of O. sativa under LN conditions, especially in Myanmar and China (Fig. 5g right). We also calculated the nucleotide diversity within an ~1.6 Mb interval surrounding the gene and observed an interval of ~400 kb surrounding OsNPF6.1 with significantly reduced nucleotide diversity in OsNPF6.1 HapB rice relative to OsNPF6.1 HapX rice using Rice3K data (Fig. 5h ) [25] . This selective sweep is consistent with other reported regions associated with low nucleotide diversity and artificial selection in rice [26] . LN treatment rapidly induced the expression of OsNPF6.1 (Supplementary Fig. 18 ). This LN induced expression pattern of OsNPF6.1 HapB was confirmed by the promoter: reporter assay (Supplementary Fig. 18b ). Under LN condition, the basal promoter activity of OsNPF6.1 HapB without OsNAC42 expression (as of vector treatment YFP-alone) was about three folds of that of OsNPF6.1 HapA at low nitrate condition (0.2 mM) (Supplementary Fig. 18c ). By contrast, under high nitrate condition (1 mM and 5 mM), the basal promoter activity between OsNPF6.1 HapB and OsNPF6.1 HapA was significant only when co-expression of OsNAC42 could activate the promoter activity of OsNPF6.1 HapB , but not that of OsNPF6.1 HapA (Supplementary Fig. 18d, e ). The transactivation activity of OsNAC42 on OsNPF6.1 HapA could only be observed at HN condition (5 mM) (Supplementary Fig. 18e ). With the same reporter system but treatment of various N concentrations, we further found that OsNPF6.1 HapB promoter was more active at as low as 0.2 mM KNO 3. Low KNO 3 (0.2 mM) content could activate promoter activity of OsNPF6.1 HapB and higher (10 mM) level even represses OsNPF6.1 HapB promoter activity. That means the OsNPF6.1 HapB promoter could sense the cellular level of NO 3 − and responses to environmental N deficiency condition. We found significant interaction between the two genes in the core population (Supplementary Fig. 19 ). The cultivars Suwon264, Kexuan13, and IR36 harboring OsNAC42 or OsNPF6.1 elite alleles, showed greater NUE phenotypes than those harboring no elite alleles (Supplementary Fig. 20a ). OsNPF6.1 was genetically distant to other published NPF6 subfamily genes though it belonged to rice NPF6 gene clade (Supplementary Fig. 20b ), while OsNAC42 was genetically close to NAC16 and not related to other NACs (Supplementary Fig. 20c ). In the Rice3K database ( http://snp-seek.irri.org/ ) [27] , there are 209 varieties harboring OsNPF6.1 HapB , accounting for only 9.7% of the total (Fig. 5i ), while 1302 varieties (43.01%) harbor the OsNAC42 HapC allele (Supplementary Fig. 20d ). Therefore, OsNPF6.1 HapB is a rare elite allele utilized in rice breeding. We further evaluated its breeding potential for yield. The yield per plot in both HN and LN fields (Fig. 5j, k ) and NUE (Fig. 5l ) of OsNPF6.1-D1 (gain-of-function T-DNA insertion line) and OsNPF6.1 HapB overexpression line were increased, while those of OsNPF6.1 HapA knock-out line decreased. It indicates overexpression of OsNPF6.1 HapB confers a high NUE, and the elite allele OsNPF6.1 HapB is highly beneficial in efforts to enhance NUE and yield in rice. Plant NUE is inherently complex trait. In this study, based on a large data set of NUE-traits collected from three successive years of field experiments, we integrated the GWAS approach with a series of functional characterizations of rice NUE genes, leading to the identification of a nitrate transporter OsNPF6.1 and a transcription factor OsNAC42, which directly regulates the transcription of OsNPF6.1 . This large scale of field work has never been carried out in any other GWAS studies. Therefore, our work represents a large genomic study in agriculture genomics as field trailed GWAS is more realistic and more competent for identifying genes improving rice NUE in field. More importantly, we identified OsNPF6.1 HapB , a rare variant of OsNPF6.1 that improves NUE by increasing rice EPN and YPP. Strikingly, the elite haplotype OsNPF6.1 HapB changed the sequences of both the encoded protein and promoter elements. Further, we established that the elite haplotype OsNPF6.1 HapB was transactivated by OsNAC42 to regulate nitrate uptake. We show that OsNPF6.1 and OsNAC42 are two genes in improving NUE in cultivated rice. Our genetic evidence also revealed that OsNAC42 transcriptionally regulated OsNPF6.1 HapB (Supplementary Fig. 21 ). The co-expression pattern of OsNAC42 and OsNPF6.1 in response to altered nitrogen concentrations also suggested they might act a signaling module in the NUE network. Notably, elite allele OsNPF6.1 HapB has been lost in 90.3% of rice varieties, probably due to the increased usage of nitrogen fertilizer over past decades [28] . From GWAS analysis of 3-year field test, we identified a haplotype of OsNPF6.1 , OsNPF6.1 HapB , that contributes to high NUE and yield under LN condition. Importantly, this elite haplotype contains not merely a single SNP variation (178766 bp) in OsNPF6.1 coding sequence which leads to 160 Gly to Asp, and more OsNAC42 transactivating sites on the promoter region of OsNPF6.1 . We have revealed that the SNP variation leads to the increased transport activity of OsNPF6.1, whereas the increased binding sites in its promoter enable a strong transactivation of OsNAC42 on its expression. We further confirmed the critical role of this elite haplotype by constructing transgenic overexpression and CRISPR/Cas knock-out lines, which improved and reduced the NUE and yield, respectively. Thus, our study identified an elite haplotype of a nitrate transporter, and revealed the mechanism how the genetic variations contribute to NUE. Compared with known nitrate-transporter genes such as OsNRT1.1A , OsNRT1.1B , and OsNRT2.3 [7] , [8] , [9] , the OsNPF6.1 HapB functions as a unique effective nitrate transporter under low nitrate condition based on following evidences. OsNPF6.1 is localized in the plasma membrane (Supplementary Fig. 7a ), and is highly expressed in root cells (Supplementary Fig. 8b, c, f ), thus could be enable to activate N uptake and signaling pathways under LN condition. More importantly, OsNPF6.1 HapB promoter was more active at as low as 0.2 mM KNO 3 , different from other known nitrate transporters including OsNRT1.1B. Meanwhile, distinguished from the other transcription factors related with NUE (e.g., OsGRF4), the transcription factor OsNAC42 trans-regulates OsNPF6.1 and other possible genes related with NUE. In summary, we demonstrate that nitrogen transporter OsNPF6.1 HapB , trans-regulated by transcription factor OsNAC42, confers NUE by activating nitrate uptake in rice. These genes will accelerate future efforts aimed at NUE, yield and grain quality improvement of rice through the approaches of transgenics, marker-assisted selection, and genome editing. Plant materials The seeds of 461 accessions were collected, stored, and supplied by State Key Laboratory of Crop Genetics and Germplasm Enhancement, Nanjing Agricultural University, China. We measured the NUE-related agronomic traits of PH, EPN of the 461 lines grown in LN and HN fields in the year 2014. A total of 117 rice accessions were selected for NUE evaluation in the study with extreme N-related phenotypes in HN and LN. All the materials were planted in the field at the experimental farm of Nanjing Agricultural University, Nanjing, China. For field experiments, the accessions were grown in a completely randomized block design with four replicates. The field experiments were carried out as a randomized block design with two N levels (+N, with 300 kg/ha N fertilizer, and 0 N fertilizer) in two blocks. P and K fertilizers were applied at 100 and 100 kg/ha, respectively. There were 20 and 17 cm between rows and individuals, respectively, which were sown on 10 May and transplanted on 20 June 2014–2016. Plants of each accession were planted as well as the controls Qianzhongliang (QZL), which is tolerant to low N and Nanjing6 (NJ6), which is sensitive. We surveyed PH under high and low N conditions (PH and PHLN) and PH ratio of low N/high N (PHR); EPN under high and low N conditions (EPN and EPNLN), and EPN ratio of low N/high N (EPNR); YPP under high and low N conditions (YPP, YPPLN), and YPP ratio of low N/high N (YPPR). PHR and EPNR, key determinants for rice growth and development, were chosen as the indices of low N tolerance [29] . In addition, we evaluated YPPR for yield index of low N tolerance. NIL lines NIL(HapA) and NIL(HapB) were derived from CSSLs (BC 6 F 4 ) of Guichao2 and donor parent Koshihikari. A ~3.8 K (consisting of ~2 K upstream sequence and entire OsNPF6.1 gene) fragment was amplified and cloned into the pCUbi1390 vector to construct the complementary line (Nip pHapB::NPF6.1 HapB ). The T-DNA mutant 4A-03841L ( OsNPF6.1-D1 ) was obtained from RiceGE in Korea. The T-DNA insertion was verified using primers located in the pGA2715 vector and the promoter and CDS of OsNPF6.1 . The overexpression lines were constructed with the entire OsNPF6.1 gene CDS and the pCUbi1390 vector (maize Ubiquitin promoter) and three independent lines were selected for further study. The OsNPF6.1Pro :GUS lines were constructed with the entire OsNPF6.1 gene promoter (~2 K upstream sequence of OsNPF6.1 CDS) and the pCAMBIA1381Z vector. The tilling mutant ( osnac42 ) was obtained from the Crop Tilling mutant database of Prof. Chunming Liu, Key Laboratory of Plant Molecular Physiology, CAS ( http://www.croptilling.org ) [30] . The full-length gene of OsNAC42 in the tilling mutant was amplified and sequenced using an ABI3730xl DNA sequencer, following standard protocols. Relevant primer sequences were listed in Supplementary Data 2 . Sequencing and genotype imputation Genomic DNA was extracted from leaf tissues of the 117 rice accessions using the DNeasy Plant Mini Kit (Qiagen, Germany). A restriction site-associated DNA sequencing (RAD-Seq) library was prepared for single end-sequencing according to Tang et al. [19] . with some modifications. Briefly, barcodes were 6-bp long, being at least two mutational steps separated from each other. Two microgram of genomic DNA from each inbred were digested for 1 h at 37 °C in a 50 μL reaction with 50 U of Eco RI (New England Biolabs). The RAD library was sequenced on an Illumina Hiseq2500. The raw reads of high quality were assembled based on the genomic sequences of the japonica rice cultivar. Nipponbare using TMAP3.6. Parameters were set as default to classify whether mismatches were sequencing errors or genomic variants. Reads were separated by barcode and trimmed at the 3′ ends. SNPs of each sample were collected using the TASSEL pipeline [31] . Filtering and imputation were performed to call the first 64-bp of the high-quality reads. LD decay was calculated with PopLDdecay software [32] . The SNP cladogram-tree dataset was generated using the neighbor-joining method as provided in TASSEL [33] . We downloaded the core collection of 3023 sequenced rice genomes with 6,572,189 filtered single nucleotide variations (SNVs) from the Rice3K sequencing project ( http://snp-seek.irri.org/ [27] ). To select tag SNPs, PLINK [34] was used to calculate linkage disequilibrium (LD) between each pair of SNPs within a sliding window of 50 SNPs and we removed all but one SNP that were in perfect LD (LD = 1). The remaining SNPs were regarded as tag SNPs. We used PLINK for further quality control (QC) by removing SNVs with MAF < 0.05 and excluding rice genomes with more than 10% missing genotypes [34] . Totally, 6,550,965 variants and 2, 901 rice genomes passed the filters and QC. Beagle 4.0 was used to impute the missing SNVs in the reference rice genomes. We used SHAPEIT2 to firstly infer the haplotypes among the set of genotypes studied [35] . We used the reference panel of inferred haplotypes at a dense set of SNPs to impute into the individuals that were genotyped at a subset of the SNPs by IMPUTE2 software [36] . We used the info metric (cutoff = 0.70) to remove poorly imputed SNPs from the imputed genotypes. We finally identified a total of 1,531,224 SNPs in the core population for GWAS through genotyping by sequencing and imputation after removing nucleotide variations with missing rates > 0.2 and minor allele frequency < 0.05. Association analysis The number of subpopulations (K) was determined using STRUCTURE version 2.3.4, and each accession was assigned to a subpopulation with the membership value ( Q value) > 0.5 [37] , [38] . Population structure matrix Q was calculated using STRUCTURE. Kinship matrix K was computed using the TASSEL 2.1 [39] . As no obvious difference was observed among the five subpopulations (Supplementary Fig. 2f ), we applied general linear model rather than mixed linear model to avoid over-fitting. Real-time PCR To investigate expression of the NUE-related genes, total RNA was isolated using plant RNA purification reagent (Invitrogen). Real-time PCR was done in a real-time PCR machine (I-Cycle, BioRad), with each reaction containing 200 ng of first-strand cDNAs, 0.5 μL of 10 mmol L-1 gene-specific primers, and 12.5 μL of real-time PCR SYBR MIX (iQ ™ SYBR ® Green Supermix, Bio-Rad). Amplification conditions were 95 °C for 5 min followed by 40 cycles of 95 °C for 15 s and 60 °C for 60 s. The rice Actin1 gene was selected as the endogenous reference. The PCR specificity was examined on 3% agarose gels using 5 μL from each reaction to check for the correct product length and make sure there were no primer dimers or nonspecific amplicons. The primers for real-time PCR together with cDNA amplification were listed in Supplementary Data 2 . Subcellular localization For the subcellular localization of the OsNPF6.1 and OsNAC42 protein in rice protoplasts, the first 645 bp of the OsNPF6.1 coding sequence were amplified and inserted into the Xba I and Bam HI sites of the pAN580 vector while the last 1176 bp of the OsNPF6.1 coding sequence were amplified and inserted into the Bgl II and Pst I sites of the pAN580 vector. The full OsNAC42 coding region was amplified and inserted into the Bgl II and Pst I sites of the pAN580 vector. The transient expression constructs were transformed into rice protoplasts which were isolated from 2-weeks seedlings [40] . After 16 h incubation, the GFP fluorescence was observed using a confocal laser scanning microscope (Leica TCS SP5). Relevant primer sequences were given in Supplementary Data 2 . Determination of nitrate influx rate using 15 NO 3 − NILs (HapA and HapB), ZH11 and osnac42 mutant were grown in IRRI nutrient solution [41] for 3 weeks. Uniform seedlings were chosen for further treatments. The seedlings were grown in solution without N for 4 days, then transferred to 0.1 mM CaSO 4 for 1 min and treated with 0.125 or 1.25 mM Ca( 15 NO 3 ) 2 for 60 or 5 min, respectively. Finally, the seedlings were returned to 0.1 mM CaSO 4 for 1 min for nitrate influx rate determination using 15 NO 3 − . Functional analysis of OsNPF6.1 in Xenopus oocytes OsNPF6.1 haplotypes ( OsNPF6.1 HapA and OsNPF6.1 HapB ) were expressed in Xenopus oocytes and a two-electrode voltage-clamp was used to record currents. Full-length OsNPF6.1 HapA and OsNPF6.1 HapB coding sequences and the expression vector pT7TS were treated by Bgl II and Not I, and purified by AxyPrep™ PCR Cleanup kit. Then purified products were subcloned into the expression vector pT7TS [7] , [42] . The correct plasmid DNA was extracted and Eco RI was used to linearize the DNA, followed by phenol/chloroform extraction and ethanol precipitation. Complementary RNAs (cRNAs) were synthesized with the mMESSAGE mMACHINE T7 transcription kit (Invitrogen, Thermo Fisher Scientific). Transcripts were dissolved in nuclease free water at a final concentration of 2 μg/μL and stored at −80 °C prior to use. X. laevis oocytes were isolated in 25 mL modified washing buffer (NaCl 96 mM; KCl 2 mM; MgCl 2 5 mM; and 5 mM HEPES; pH 7.4 adjusted with NaOH) containing 43 mg collagenase and 12.5 mg trypsin inhibitor for 65 min, and then stored in Ringer’s buffer (NaCl 96 mM, KCl 2 mM, MgCl 2 5 mM, CaCl 2 0.8 mM and HEPES 5 mM, pH 7.4) supplemented with 5% dialyzed horse serum, 50 µg/mL tetracycline, 100 µg/mL streptomycin and 550 µg/mL sodium pyruvate at 4 °C for overnight. Oocytes were injected with 27.6 nL RNA after recovery and then were incubated in NO 3 − -free MBS (Modified Barth’s Solution) (88 mM NaCl, 1 mM KCl, 2.4 mM NaHCO 3 , 0.71 mM CaCl 2 , 0.82 mM MgSO 4 , and 15 mM HEPES, pH 7.4) for 2 days. After two days, two-electrode voltage-clamp technique was applied using an OC-725C amplifier (Warner Instruments) at room temperature (20 °C). The microelectrodes were filled with 3 M KCl. For the inward currents at single nitrate concentration, oocytes were voltage-clamped at −60 mV, and the inward currents elicited by control solution (no nitrate substrate) or with 0.5 or 2.5 mM NO 3 − at pH 5.5. For the current–voltage ( I – V ) curve measurement, the oocyte was clamped at −60 mV and assayed from −20 to −120 mV in 20 mV step for 300 ms each. The OsNPF6.1 HapA or OsNPF6.1 HapB -injected oocyte was exposed to 10 mM nitrate at pH 5.5 and pH 7.4, respectively. Data acquisition and analyses were carried out with Digidata 1440 A and PCLAMP10.2 software (Axon Instruments Inc., Union City, CA, USA). Oocytes injected with water were used as the negative control. Relevant primer sequences were listed in Supplementary Data 2 . Nitrogen and nitrate concentration assays The nitrogen concentration of leaves in LN and HN was determined as Kjeldahl nitrogen using a Gerhardt device. N concentration = c ( V − V 0) × 0.014 × D × 1000 / m . c (H 2 SO 4 standard solution) = 0.02 mol/L; V is the volume of H 2 SO 4 standard solution used in the sample; V 0 is the volume of H 2 SO 4 standard solution used in blank; D is the separation multiple, constant volume/separated volume; and m is the sample quantity. The tillering nodes were sampled when tillering nodes occurred. Nitrate concentration was determined on a continuous-flow autoanalyzer (Autoanalyzer3, Bran & Luebbe). Every sample had three replicates. EMSA EMSA was performed with a Light Shift Chemiluminescent EMSA Kit (Thermo Scientific) according to the manufacturer’s instructions [43] . Probes of OsNPF6.1 HapA and OsNPF6.1 HapB promoter haplotypes were labeled by PCR with 5′ biotin-labeled primers listed in Supplementary Data 2 . Short oligonucleotide sequences containing CACG motifs were directly synthesized as biotin-labeled probes. Unlabeled DNAs (100-fold excess of labeled probes) were used as competitors in this study. The MBP (Maltose Binding Protein) fusion proteins MBP-OsNAC42 and MBP-OsNAC42M were separately purified using amylose resin (New England Biolabs, E8021S) beads according to the manufacturer’s instructions [44] . Chromatin immunoprecipitation The ChIP assay was adapted from Zhao et al. [45] . Total DNA of three-week-old seedlings of Nipponbare rice was extracted. The total DNA was sheared into 100–500 bp fragments using an ultrasonic crusher. E.coli expressed MBP-OsNAC42 and MBP-OsNAC42M proteins were purified. MBP-OsNAC42, MBP-OsNAC42M and sheared rice DNA fragments were co-incubated with amylase Resin (NEB, E8021S, MBP beads) for 8 h. The incubation buffer included: 140 mM NaCl, 2.7 mM KCl, 10 mM Na 2 HPO 4 , 1.8 mM KH 2 PO 4 , 1% methanol. After 8 hours co-incubation, 125 mM glycine was further added into the beads mixture and incubated for 10 min. MBP beads were washed three times using incubation buffer. For each of 400 ml volume of the samples, add 16 μL 5 M NaCl and was incubated for another 8 h to breakdown associated DNA with MBP-OsNAC42 and MBP-OsNAC42M proteins. Subsequently, DNA fragments were extracted using the phenol–chloroform method for further ChIP-qPCR analysis with a Bio-Rad CFX96 real-time PCR detection system. PCR were performed in triplicate for each sample, and the expression levels were normalized to the input sample and only MBP control treatment for enrichment detection. The enrichment folds were calculated against the amount of bound DNA of rice ubiquitin promoter. Relevant primer sequences were given in Supplementary Data 2 . Luciferase assays N. benthamiana leaves were agro-infiltrated with Agrobacterium tumefaciens EHA105 strains carrying the various combinations of DNA construct ( OsNPF6.1 HapA : luc , OsNPF6.1 HapB : luc ). Leaves of N. benthamiana were harvested after 48 h infiltration and luciferase activity was assayed [46] . N. benthamiana leaves were kept in dark for 5 min after adding 1 mM luciferin to quench the fluorescence. Quantitative LUC activity was determined by Microplate Luminometer (Promega). Relevant primer sequences were given in Supplementary Data 2 . Selective sweep analysis A haplotype network construction of OsNPF6.1 was generated using PopART version 1.7 [47] . DnaSP version 4.0 [48] was used to calculate total nucleotide diversity per nucleotide site ( π ), relative ratio of π , and selective sweep signals [26] , [49] . Reporting summary Further information on research design is available in the Nature Research Reporting Summary linked to this article.